Casimir-like forces at the percolation transition Percolation and critical phenomena show common features such as scaling and universality. Colloidal particles, immersed in a solvent close to criticality, experience long-range effective forces named critical Casimir forces. Building on the analogy between critical phenomena and percolation, here we explore the possibility of observing long-range forces near a percolation threshold. To this aim, we numerically evaluate the effective potential between two colloidal particles dispersed in a chemical sol, and we show that it becomes attractive and long-ranged on approaching the sol percolation transition. We develop a theoretical description based on a polydisperse Asakura–Oosawa model that captures the divergence of the interaction range, allowing us to interpret such effect in terms of depletion interactions in a structured solvent. Our results provide the geometric analogue of the critical Casimir force, suggesting a novel way for tuning colloidal interactions by controlling the clustering properties of the solvent. Effective interactions have an important role in the physics of colloidal dispersions [1] . A notable example is provided by depletion interactions, that is, interactions arising from the presence of a cosolute (for example, polymers and surfactants) in the suspension. The pioneering works by Asakura–Oosawa (AO) and Vrij [2] , [3] have shown that, when two hard-sphere (HS) colloids are immersed in a solution in the presence of small cosolute particles, the latter are excluded from the available volume between colloids when the two are closer than the cosolute typical size. As a result, a net entropy-driven depletion attraction arises. In general, the strength and the range of the depletion attraction can be tuned by modifying the cosolute concentration and size. Depletion interactions have thus far mostly been exploited for monodisperse cosolutes, such as non-adsorbing polymers or HSs, generating short-range effective forces. A solvent composed by cosolutes of different size could introduce a structure in the effective potential controlled by the different cosolute length scales [4] . Interestingly, if the cosolutes are constituted by a chemical sol (that is, a sol composed by particles linked into clusters through irreversible bonds) close to its percolation locus, all length scales will enter in V eff , but in a scale-free mode. Indeed, when the percolation threshold is approached from the sol phase, the cluster size distribution follows a universal power-law dependence and clusters of all sizes are present (up to a cutoff that is function of the distance from percolation). Thus, it is legitimate to ask whether two colloids, immersed in a sol of clusters close to percolation, experience a long-ranged effective force, whose characteristic length scale diverges at percolation. This question becomes even more interesting if we consider the analogy between percolation and thermal critical phenomena. Percolation theory describes the growth of clusters in a system on approaching the percolation threshold, the point at which an infinite spanning cluster appears [5] . Similarly, the theory of critical phenomena describes the growth of correlated regions on approaching a second-order critical point, where the size of the correlated regions diverges [6] . Clusters of different sizes in percolation have the same role as the thermal critical fluctuations close to the second-order critical point [7] , both being described by scale-free distributions, whose first moment shows a power-law behaviour approaching the transition. Both the connectivity length in percolation and the correlation length in critical phenomena diverge at the transition. It is well known that colloidal particles immersed in a solvent that is close to a second-order critical point experience long-range effective forces. These forces originate from the confinement of the solvent critical fluctuations between the surfaces of distinct colloids [8] . The (universal) resulting effective potential decays with an exponential law controlled by the thermal correlation length of the solvent, diverging at the critical point [8] , [9] . These forces, named as critical Casimir forces for their analogy with the Casimir effect occurring when the electromagnetic field is confined between two metal surfaces, have been measured in recent experiments [10] . Owing to their universal nature, critical Casimir interactions do not depend on the specific properties of the solvent but only on the geometry of the confining surfaces and on their ability to absorb the solvent (boundary conditions), giving rise to both attractive or repulsive interactions [11] , [12] , which have been exploited to induce colloidal aggregation [13] , [14] , [15] , [16] , [17] , [18] , [19] , [20] . It has also been conjectured that proteins in membranes of living cells experience weak long-range critical Casimir forces [21] . As percolation shares scaling and universality with critical phenomena, we may expect a mechanism analogous to the critical Casimir effect to take place when colloidal particles are immersed in a sol close to its percolation threshold. Here we show that indeed a long-range force, created by confining the fluctuations of the cluster sizes, develops between colloids, and that its interaction range is controlled by the sol connectivity length ξ . The resulting effective potentials are compatible with the picture of depletion induced by a polydisperse system. To this aim, we perform simulations of two colloidal particles immersed in a chemical sol close to its percolation point. Fixing the total packing fraction occupied by the clusters, we explore different distances from percolation, that is, cluster size distributions with different cutoff. Our results provide evidence that the analogy between percolation and critical phenomena can be exploited to induce novel kind of effective forces between colloidal particles, which are controlled by the clustering properties of the solvent. Effective potentials in a sol close to percolation We perform Monte Carlo (MC) simulations to evaluate the effective potential V eff between two HS colloids of diameter σ c immersed in a fluid composed of clusters. Clusters are made by N =10,836 HS monomers of size σ m =0.1 σ c , randomly connected with a maximum functionality of three (as described in the Methods section) and are treated as rigid objects, which are allowed to translate and rotate, interacting between themselves and with the two colloids via excluded volume repulsion only. Consistent with the hypothesis of a chemical sol (irreversible bonds), clusters do not break nor coalesce. The total cluster packing fraction is fixed to ϕ =0.052, whereas the distance to the percolation transition (and the associated cluster distributions) changes. In simulations, the distance from the transition is controlled by measuring the fraction p of formed bonds [5] . p is the analogous of the temperature in critical phenomena and its critical values at the percolation threshold is indicated with p c . Snapshots of the system at different p are shown in Fig. 1 . 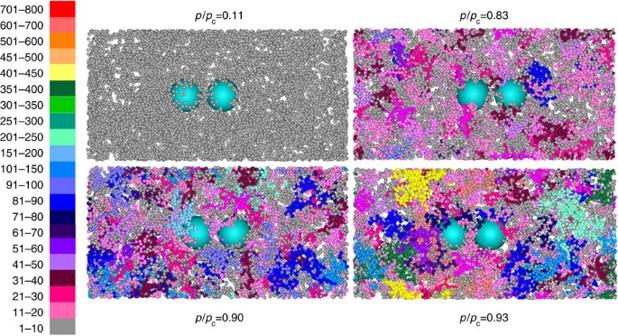Figure 1: Clustering of the sol close to percolation. Snapshots of the system for differentp, withp→pc. Each snapshot shows the two colloids immersed in the sol of clusters on approaching the percolation treshold. Clusters of different sizes are represented in a different colour (see legend). Figure 1: Clustering of the sol close to percolation. Snapshots of the system for different p , with p → p c . Each snapshot shows the two colloids immersed in the sol of clusters on approaching the percolation treshold. Clusters of different sizes are represented in a different colour (see legend). Full size image We have generated, as described in the Methods section, cluster distributions for different values of p for p → p c . For each selected p , we also evaluate the connectivity length ξ defined as [5] , where n ( s ) is the number of clusters of size s (with the constraint = N ), and R s is the radius of gyration of a cluster composed of s monomers with positions : R s =[(1/2 s 2 ) ] 1/2 . In the course of the MC simulation, the volume around the two HS colloids is explored by clusters of different size. Hence, the two colloids experience around them the presence of different clusters that fluctuate in size. Such fluctuations are analogous to the critical density fluctuations in the critical Casimir effect, and are responsible of the emergence of a long-range force when confined between the surfaces of the two colloids. 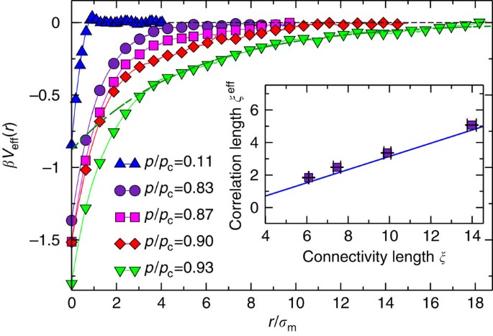Figure 2: Effective potentials between two colloids in a sol of clusters. Evolution of the effective potentialVeffon approaching the percolation threshold at fixed sol packing fractionϕ=0.052.ris the surface-to-surface distance between the two colloids. The thick line shows a typical exponential fit to the data in the intervalr/σm>3, which is used to estimate the correlation lengthξeff. Inset: correlation lengthξeffextracted fromVeff(squares) against the connectivity length defined in Equation (1), both in units ofσm. Errors on thex-andyaxis are, respectively, the standard error in evaluating the connectivity length over several configurations, and the standard error in performing the exponential fit for extracting the correlation length. The latter is of the order of 1%. The solid line is calculated using the theoretical modelling proposed in Equation (6). The linear relation suggests thatVeffdiverges with the same power-law ofξat the percolation transition. Figure 2 shows the evolution of the effective potential for different p , exploring the range from p / p c ≈0.1 to p / p c ≈0.93. For p / p c >0.8, the system is sufficiently close to percolation to sample the universal features of n ( s ) (as explained in the Methods section). To probe values of p / p c >0.93 would require prohibitively larger simulation boxes. Far from percolation, when the sol is mainly composed of monomers, we recover the depletion potential between two colloids immersed in a HS fluid [22] , [23] and V eff shows a typical oscillatory behaviour, whose characteristic length scale is controlled by the monomer size. On increasing p , V eff turns completely attractive and the interaction range becomes longer and longer. The long-distance behaviour is well described by an exponential decay exp(− r / ξ eff ), the same functional form that applies to the critical Casimir potential. To show that the interaction range is controlled by the connectivity length of the sol, we compare the correlation length ξ eff , extracted from the exponential fit modelling the decay of V eff , with the connectivity length ξ of the sol (Equation (1)) in the inset of Fig. 2 . For all investigated P values, we find a linear relation between ξ and ξ eff , reinforcing the hypothesis that, close to percolation, the range of V eff is indeed related to the typical size of the clusters composing the sol. Figure 2: Effective potentials between two colloids in a sol of clusters. Evolution of the effective potential V eff on approaching the percolation threshold at fixed sol packing fraction ϕ =0.052. r is the surface-to-surface distance between the two colloids. The thick line shows a typical exponential fit to the data in the interval r / σ m >3, which is used to estimate the correlation length ξ eff . Inset: correlation length ξ eff extracted from V eff (squares) against the connectivity length defined in Equation (1), both in units of σ m . Errors on the x- and y axis are, respectively, the standard error in evaluating the connectivity length over several configurations, and the standard error in performing the exponential fit for extracting the correlation length. The latter is of the order of 1%. The solid line is calculated using the theoretical modelling proposed in Equation (6). The linear relation suggests that V eff diverges with the same power-law of ξ at the percolation transition. Full size image To provide evidence that the long-range phenomenon originates from the connectivity properties of the sol, we calculate—for p / p c ≈0.93—the effective potential for a system with the same cluster size distribution, but in which bonds are reversible and clusters break and reform in time. This corresponds to select an energy scale for the bond interaction and a temperature for which in equilibrium, the same fraction of bonds among cosolute monomers is present (see Methods). A comparison between V eff ( r ) calculated for reversible and irreversible bonds is shown in Fig. 3a . We notice the dramatic effect of the finite bond lifetime on the range of the effective potential: when clusters are reversible, the potential is attractive only up to a few monomer sizes. In order to provide further evidence that the connectivity length controls V eff at large distances, we show in Fig. 3b the comparison between V eff for p / p c =0.93 calculated, respectively, at ϕ =0.052 (as in Fig. 2 ) and at ϕ =0.105. As p / p c is the same in the two cases, the sol is characterized by the same cluster distribution (see Methods), and hence by the same ξ . We find that the long-distance part of the potential is well described by an exponential function having the same decay length for both values of the sol packing fraction, supporting the possibility of an universal behaviour at large distances. 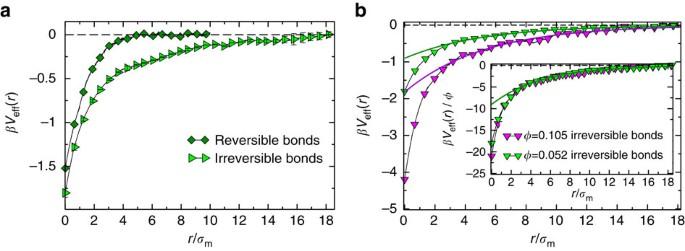Figure 3: Role of the lifetime of sol clusters and of sol packing fraction. (a) Effective potential between two HS colloids in a solution of particles that forms reversible (diamonds) and irreversible bonds (triangles), with the same cluster size distribution atp/pc=0.93 andϕ=0.052. The irreversible potential is averaged over two different realizations of the cluster fluid. Error bars for this potential are calculated from the difference of the two realizations, finding that forr/σm<15 the error does not exceed 5% of the estimated value. (b) Comparison of the investigated effective potentials generated by irreversible clusters at two different packing fractions along an iso-pline (see Methods). Full lines are exponential fits of the long-range tail ofVeff. The best fit decay length is ≈5σmforϕ=0.052 and ≈5.3σmforϕ=0.105. The inset shows that the long-distance parts of the potentials superimpose within numerical error when the two potentials are scaled by the packing fraction. Figure 3: Role of the lifetime of sol clusters and of sol packing fraction. ( a ) Effective potential between two HS colloids in a solution of particles that forms reversible (diamonds) and irreversible bonds (triangles), with the same cluster size distribution at p / p c =0.93 and ϕ =0.052. The irreversible potential is averaged over two different realizations of the cluster fluid. Error bars for this potential are calculated from the difference of the two realizations, finding that for r / σ m <15 the error does not exceed 5% of the estimated value. ( b ) Comparison of the investigated effective potentials generated by irreversible clusters at two different packing fractions along an iso- p line (see Methods). Full lines are exponential fits of the long-range tail of V eff . The best fit decay length is ≈5 σ m for ϕ =0.052 and ≈5.3 σ m for ϕ =0.105. The inset shows that the long-distance parts of the potentials superimpose within numerical error when the two potentials are scaled by the packing fraction. Full size image Generalized AO model for a polydisperse depletant To gain a deeper insight in the mechanism that controls the range of V eff close to percolation in a chemical sol, we now develop a theoretical framework based on the analogy with depletion interactions. When small depletant particles are added to a colloidal suspension, an attractive entropic force between colloids builds up, because of the exclusion of the depletant from the region between particles when their relative distance is comparable or smaller than the depletant diameter [1] . In the venerable AO–Vrij model [2] , [3] , introduced to describe the effective interactions between colloids in a solution of non-interacting polymers, depletants are modelled as an ideal gas that interacts via hard-core repulsion with the HS colloids only. In the case of monodisperse depletant particles of radius R , the AO effective potential between two HS colloids at a surface-to-surface distance r and depletant number density ρ is where the Θ function indicates that the potential vanishes for distance longer than 2 R . We propose to model the sol close to percolation as a polydisperse HS system distributed according to the cluster size distribution n ( s ). Each cluster is represented as a sphere of radius R s , the cluster gyration radius, reducing the problem to that of two colloids immersed in a sea of ideal depletant particles of different size. Following AO, clusters interact only with the colloids via a hard-core repulsion. As σ m is significantly smaller than σ c only very close to percolation the largest cluster size becomes comparable to the colloid size. Apart from this small region, the depletion hypothesis is valid [24] . Close to percolation, the cluster size distribution n s assumes the universal form [5] , [25] where τ =2.18 is a critical exponent (in the random-percolation universality class) and s c controls the exponential cutoff of the power-law distribution, approaching infinity at percolation. Moreover, Γ( x , y ) is the incomplete Γ function entering via the normalization condition sn ( s )d s = N . Summing overall clusters, the resulting potential is βV AO ( r , R s , n ( s )/ V )/d s V , where V is the volume. Building on the universal properties of the clusters shape close to percolation [5] , it is possible to relate the number of monomers s in the cluster to R s via the fractal exponent D , whose universal value (in random percolation theory) is D =2.53, Hence, the total potential becomes, where ρ 1 is the monomer number density and the lower integration limit in Equation (5) accounts for the Θ function in each AO contribution. This indicates that only clusters with diameter larger than r participate in building β ( r ). Finally, integrating over the cluster size we obtain, This functional form depends on the percolation exponents and, for large r , its asymptotic behaviour is To compare the theoretical predictions based on the AO approach with the effective potential previously calculated, we first verify that the clusters size distribution and the cluster gyration radius used in the MC simulations are consistent with the scaling laws predicted by percolation theory and extract the corresponding s c value. 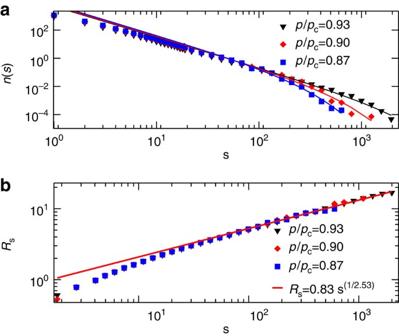Figure 4: Clustering properties of the sol: (a) Cluster size distributionn(s) of the sol used in MC simulations and (b) radius of gyrationRsas a function of the cluster sizesfor differentp, withp→pc. Lines inaare power-law fits ton(s) modulated by an exponential function, according to Equation (3). The solid line inbis a fit toRsfollowing Equation (4). The resulting fit valuesscandR1are used for evaluating the effective potential in Equation (5). Note that a theoretical description based on universal properties of cluster fluids close to percolation applies only for cluster sizes above 50. Figure 4 shows n ( s ) and R s with respect to the theoretical predictions of Equation (3) and Equation (4). For clusters larger than 50 monomers, the model-independent scaling laws properly describe the data, suggesting that for r >2 R s =50 , theoretical predictions can be meaningfully compared with the effective potentials calculated from MC simulations. Figure 4: Clustering properties of the sol: ( a ) Cluster size distribution n ( s ) of the sol used in MC simulations and ( b ) radius of gyration R s as a function of the cluster size s for different p , with p → p c . Lines in a are power-law fits to n ( s ) modulated by an exponential function, according to Equation (3). The solid line in b is a fit to R s following Equation (4). The resulting fit values s c and R 1 are used for evaluating the effective potential in Equation (5). Note that a theoretical description based on universal properties of cluster fluids close to percolation applies only for cluster sizes above 50. Full size image The resulting potentials for different p are reported in Fig. 5 . A surprisingly good agreement between MC results and the theoretical model is found for r >2 R s =50 ~7.8 σ m , confirming that the effect of the sol can be modelled as a depletion interaction acting on all length scales associated with the clusters. We also extract a characteristic decay length of ( r ), using an exponential fit similarly to what done for the numerical MC data. This can be used to build a relation with ξ , yielding the curve reported in the inset of Fig. 2 , which closely follows the MC simulation results. The self-similar nature of the cluster size distribution and its widening on approaching percolation do control the interaction range. 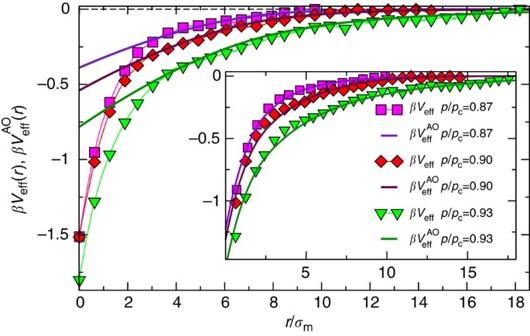Figure 5: Comparison between simulations and theory: symbols correspond toVeffextracted from simulations while solid lines arecalculated from Equation (5). As universal features of the pre-percolating fluid appear only for clusters larger than 50 monomers (Fig. 4), theoretical and numerical results show a good agreement only for distancesr>2Rs=50. Inset: comparison betweenVeff(symbols) extracted from simulations and(solid lines) obtained by repeating the calculation of the effective potential of Equation (5), in which the exact cluster size configurations used in simulations are used. Including the gyration radius of each cluster in the expression ofallows us to compare theoretical and numerical results also in the regionr<2Rs=50. Figure 5: Comparison between simulations and theory: symbols correspond to V eff extracted from simulations while solid lines are calculated from Equation (5). As universal features of the pre-percolating fluid appear only for clusters larger than 50 monomers ( Fig. 4 ), theoretical and numerical results show a good agreement only for distances r >2 R s =50 . Inset: comparison between V eff (symbols) extracted from simulations and (solid lines) obtained by repeating the calculation of the effective potential of Equation (5), in which the exact cluster size configurations used in simulations are used. Including the gyration radius of each cluster in the expression of allows us to compare theoretical and numerical results also in the region r <2 R s =50 . Full size image To strengthen even more the comparison with , we have repeated the evaluation of the effective potential in Equation (5), by numerically summing over the very same cluster configurations used in simulations, associating each cluster with its own gyration radius, without resorting to the scaling laws. The resulting curves are shown in the inset of Fig. 5 . Including the exact cluster size distribution and the exact behaviour of the gyration radius makes it possible to properly capture even the region r <2 R s =50 with the simple superposition of the AO contributions. Hence, we conclude that the failure of the model for r <2 R s =50 is not related to the AO approximation, but to the non-asymptotic (model-dependent) behaviour, which is clearly visible in the size dependence of R g for small clusters in Fig. 4 . We have demonstrated that two colloids in a gel-forming solution experience an attractive effective potential, which becomes increasingly long-ranged on approaching the percolation transition. The range of the effective interaction is controlled by the connectivity length of the sol and diverges at the percolation transition. Such effective interaction originates from the confinement of the cluster-size fluctuations between the colloids surface, thus providing a new Casimir-like effect driven by the clustering properties of the sol. These results extend the analogy between the percolation transition and a second-order critical point [7] to the context of effective interactions. In the case of critical Casimir forces, the long-range attraction arises from the confinement of the order parameter fluctuations in between the colloids. When the latter are located at distances smaller than the correlation length, large-scale fluctuations are not allowed to occur between the colloids along the r -direction, giving rise to a non-zero net force. Approaching percolation, it is the cluster size distribution that becomes wider and larger and larger clusters appear. Similarly to critical fluctuations, clusters whose diameter is larger than the colloids surface-to-surface distance are excluded. The use of a simple theoretical description in which clusters are treated as non-interacting spheres has shown that the mechanism controlling the effective interactions can be assimilated to a depletion effect. We expect that the residual interaction among monomers of different clusters (that are not included in our simulations) would not affect significantly our results. In fact in the solvent cluster phase, most of the particle–particle interaction is already accounted in the formation of clusters and the only remaining relevant cluster–cluster contribution is related to exclude volume interactions. The fractal nature of the percolation clusters, which favours their interpenetration, and the small overall packing fraction of the sol help in modelling the resulting depletion potential with a theory that neglects cluster–cluster interactions (in analogy with the standard polymer depletants for which the AO model was conceived). It is interesting to note that the depletion mechanism has been also invoked as a guiding analogy for interpreting critical Casimir forces [16] , [26] , where the increase of the correlation length of the critical domains has been regarded as an increase of the size of the depleting objects. We remark that the developed AO approach is limited to the case in which the size of the largest cluster does not significantly exceed the colloidal size. Further we finally stress that the current analysis is based on a two-body description of the effective potential. In analogy with critical Casimir forces [27] , we expect that many-body effects will become relevant close to percolation when the interaction range becomes comparable to the colloid size. Exploiting the percolation transition for generating long-range effective forces opens up a new way to use self-assembly properties of the solvent (or cosolutes) for controlling interactions between colloidal particles. Differently to the case of critical Casimir forces that require tuning of the solvent properties close to one specific point (the critical point), percolation can be achieved for a variety of sol-densities. Finally, we have shown that the effective potential is long ranged only in the case of chemical sols, when bonds between monomers have an infinite lifetime. Experimental investigation of such phenomenon requires thus a chemical sol close to gelation. However, we speculate that the same results hold also in the case of reversible bonds but only in the limit in which bond lifetimes are significantly longer than the experimental time scales (that is, experiments that probe only a single sol microstate). In this perspective, with the increasing availability of self-assembling particles with specific design of interactions [28] , [29] such as gel-forming DNA tetramers [30] , we expect that the realization of these long-range effective forces could be implemented, paving the way for further manipulation of colloidal phase behaviour and dynamical arrest. Model To generate the sol of clusters, we study a model of particles interacting via the pairwise anisotropic Kern–Frenkel three-patches (3P) potential [31] . Particles are thus represented by HSs of diameter σ m with three attractive sites, located on the equator. The interaction potential between these sites is where is the vector between the centres of particles i and j , and is the unit vector from the centre of particle i to the centre of the α-patch on the surface. is a square well potential of width δ =0.119 and depth ε =1 The function G modulates the potential and depends on the reciprocal orientation of two particles: The angular width that controls the volume available for bonding is set to cos(θ max )=0.894717. A sketch of the 3P model is reported in Fig. 6a . The 3P system is a model for a physical gel, that is, it forms reversible clusters and its connectivity properties depend on the temperature T and the packing fraction ϕ . Hence, in principle, it is possible to tune T and ϕ in order to find state points with the desired number of inter-monomer bonds. The phase diagram of the model in the T - ϕ plane, characterized by the limited-valence gas–liquid phase separation [32] , is shown in Fig. 6b . Lines of constant number of bonds—that is, lines of equal bond probability (iso- p lines)—identify loci of similar sol structure. One of these lines is also shown in Fig. 6b . Along this line, the cluster size distribution is found to be the same within numerical resolution ( Fig. 6c ), confirming that the monomers are aggregated in clusters of similar polydispersity. 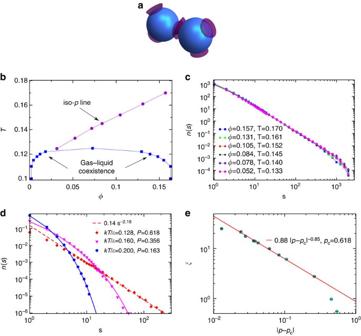Figure 6: Clustering properties of the 3P particle model. (a) Sketch of two interacting 3P particles. (b) Phase diagram of the 3P particles model showing the gas–liquid (blue squares) coexistence line and a locus of points (violet circles) of constant bond probability (p=0.565±0.010). (c) Cluster size distributionn(s) for different densities along thep~0.565 locus.n(s) is the same within the numerical precision. (d) Cluster size distribution of the Kern–Frenkel 3P model atϕ=0.052, for different temperatures (corresponding to differentp). Although at highT(p<<pc),n(s) is well described by the mean-field Flory–Stockmayer distribution (solid lines), at the percolation point (corresponding roughly tokT/ϕ=0.128),n(s) follows a power-law behaviour (dashed line) with exponentτ=2.18. (e) Connectivity lengthξof the sol atϕ=0.052 as a function of the distance from the percolation point.ξfollows a power-law behaviour with an exponent consistent with the prediction of the random percolation theory (v=0.88). Forp~pcfinite size effects appears while forp<<pc, the power-law behaviour breaks down. Herepc=0.618. The standard error in evaluating the connectivity length over several configurations is also shown. Figure 6: Clustering properties of the 3P particle model. ( a ) Sketch of two interacting 3P particles. ( b ) Phase diagram of the 3P particles model showing the gas–liquid (blue squares) coexistence line and a locus of points (violet circles) of constant bond probability ( p =0.565±0.010). ( c ) Cluster size distribution n ( s ) for different densities along the p ~0.565 locus. n ( s ) is the same within the numerical precision. ( d ) Cluster size distribution of the Kern–Frenkel 3P model at ϕ =0.052, for different temperatures (corresponding to different p ). Although at high T ( p << p c ), n ( s ) is well described by the mean-field Flory–Stockmayer distribution (solid lines), at the percolation point (corresponding roughly to kT /ϕ=0.128), n ( s ) follows a power-law behaviour (dashed line) with exponent τ =2.18. ( e ) Connectivity length ξ of the sol at ϕ =0.052 as a function of the distance from the percolation point. ξ follows a power-law behaviour with an exponent consistent with the prediction of the random percolation theory (v=0.88). For p ~ p c finite size effects appears while for p << p c , the power-law behaviour breaks down. Here p c =0.618. The standard error in evaluating the connectivity length over several configurations is also shown. Full size image In most of the work, we fix the packing fraction of the particles to ϕ =0.052, and equilibrate the system at several temperatures to probe states with different fraction of bonds p and hence different cluster size distribution. On cooling indeed the system forms larger and larger clusters, till a percolation point is reached where a spanning cluster appears. Note that 3P particles form transient clusters because of the reversibility of the bonds. To generate a model for chemical gel, after equilibration has been reached, we freeze all the bonds formed in an arbitrary configuration of the system, thereby making the clusters lifetime infinite. Once all bonds are frozen, particles belonging to different clusters cannot form new bonds and clusters behave as translating and rotating rigid objects interacting only via excluded volume among them and with the two HS colloids. This polydisperse set of clusters is then used as a chemical sol model in the numerical study of the effective potential between two colloids. Identification of the percolation threshold For the system under study (with f =3 bonding sites for each of the N particles) the fraction of bonds can be calculated from the relation p =−2‹ U ›/ Nf , where ‹ U › is the average potential energy and the factor two accounts for all the bonded sites of the system. At the percolation point ( T *, ρ *), p reaches its critical value p c . To roughly identify the percolation threshold for the 3P system at the packing fraction ϕ =0.052, we have performed MC simulations of the 3P fluid in the canonical ensemble for different temperatures T (that is, for different p ) in the absence of the two large HS colloids. The percolation point can be identified by studying the evolution of the cluster size distribution n ( s ) for different state points, which has the form of a power-law at p = p c , that is, n ( s )~ s − τ (with τ =2.18), while as p → p c n ( s ) is controlled by a scaling function, typically assumed to be exponential, that modulates the power-law (Equation (3)). The result is shown in Fig. 6d . Although at high temperatures (far from percolation), the function n ( s ) follows the mean-field Flory–Stockmayer theory [33] , [34] , at kT /ε=0.128 it is described by a power-law behaviour with the random-percolation universality class exponent [5] . Hence, for a system of N =10,836 3P particles at packing fraction ϕ =0.052, we locate to a good approximation the percolation point at kT /ε=0.128 corresponding to p c =0.618. Once p c is identified, we can study the behaviour of the connectivity length ξ defined in Equation (1), on approaching the percolation point. Close enough to the transition, random percolation theory predicts [5] that ξ follows a power-law behaviour with exponent v =0.88. Data for ξ ( p ) are shown in Fig. 6e . The power-law scaling is observed only for p / p c >0.8. For this reason, we have carried our investigation close enough ( p / p c >0.8) to the transition to observe a genuine effect associated to the incipient percolating behaviour. Numerical evaluation of the effective potential To evaluate the effective potential it is necessary to calculate P ( r ), that is, the probability that the two colloids are found at distance r . Hence, we implement an Umbrella Sampling scheme [12] , [35] that allows for a convenient parallelization of the code and to optimize the computational time by ‘flattening’ the energy barrier that can be created by the presence of large clusters and that can prevent the colloids to sample uniformly all the distances. To probe the whole distance range, we perform 40 parallel runs in which the two colloids explore 40 different windows. Hence, in the Umbrella Sampling scheme used, for each simulation the two colloids sample only a small window of distances Δ i . Each run is a standard MC simulation in the canonical ensemble, where both colloids and clusters are allowed to move with a size-dependent MC step allowing for a 30% acceptance. V eff is evaluated by constraining the two colloids to move in a window Δ i along the x axis (identifying the r -direction) of a parallelepipedal box where the length of the x -edge L x =7.6 σ c is twice the length of L y and L z . This guarantees that, for all the simulated state points, the surface-to-surface distance between colloids (and their periodic images) in all directions is always larger than the distance at which V eff goes to zero. The cluster size distribution is identical in all the 40 runs. During the single run, we evaluate the probability P ( r ,Δ i ) of finding the two colloids at a given distance r within the window Δ i . Then, the total probability P ( r ) is obtained by merging together the P ( r ,Δ i ) resulting from all the parallel runs by means of a least-squares-based algorithm. The effective potential is calculated from the relation βV eff ( r )=− In ( P ( r ))+C, where C is a constant chosen imposing V eff (∞)=0. Each potential should be averaged over several different realizations of the cluster fluid. Owing to the long computational time requested for evaluating V eff (roughly 1 month on 40 cores), our averaging is limited to two different realizations of the cluster size for each distance from the percolation threshold. How to cite this article: Gnan, N. et al. Casimir-like forces at the percolation transition. Nat. Commun. 5:3267 doi: 10.1038/ncomms4267 (2014).